Spatial segregation of polarity factors into distinct cortical clusters is required for cell polarity control Cell polarity is regulated by evolutionarily conserved polarity factors whose precise higher-order organization at the cell cortex is largely unknown. Here we image frontally the cortex of live fission yeast cells using time-lapse and super-resolution microscopy. Interestingly, we find that polarity factors are organized in discrete cortical clusters resolvable to ~50–100 nm in size, which can form and become cortically enriched by oligomerization. We show that forced co-localization of the polarity factors Tea1 and Tea3 results in polarity defects, suggesting that the maintenance of both factors in distinct clusters is required for polarity. However, during mitosis, their co-localization increases, and Tea3 helps to retain the cortical localization of the Tea1 growth landmark in preparation for growth reactivation following mitosis. Thus, regulated spatial segregation of polarity factor clusters provides a means to spatio-temporally control cell polarity at the cell cortex. We observe similar clusters in Saccharomyces cerevisiae and Caenorhabditis elegans cells, indicating this could be a universal regulatory feature. The great majority of cells are polarized, and this relies on the establishment of domains of polarity factors that occupy and confer different identity and function to restricted areas of the cell cortex. A considerable body of work has identified key polarity regulators across organisms and elucidated their mechanism of mutual recruitment, interaction and functional interdependencies in the establishment of polarity [1] . However, how polarity factors are precisely organized within cortical subdomains and how that organization relates to their function in vivo is largely unknown. Fission yeast ( Schizosaccharomyces pombe ) cells are ideally suited to study cell polarity [2] , [3] . These cylindrically shaped unicellular organisms grow and divide in a highly polarized manner. After cell division, newborn cells grow monopolarly from their ‘old end’ (existing before division) and later activate growth at their ‘new end‘, derived from the site of septation. Once cells double their original volume, they enter mitosis and bipolar cell growth stops until division is complete and growth restarts. This cyclic pattern of polarized growth activation, maintenance and inactivation relies on a hub of over 50 cortical polarity factors [2] , [3] , [4] , which accumulate at the cell ends. These include the kelch-repeat protein Tea1 and the SH3 domain-containing protein Tea4, which form part of a complex delivered to cell ends by growing microtubule tips. Once there, the Tea1–Tea4 complex is anchored to the cell end cortex by the combined action of the ERM ( E zrin- R adixin- M oesin) family protein Tea3 and the plasma membrane-associated prenylated anchor protein Mod5. Various pairwise physical interactions have been demonstrated for Tea1, Tea4, Tea3 and Mod5, suggesting that these can exist as a complex, although possibly not all simultaneously [5] . The Tea1–Tea4 complex further interacts with other polarity factors including the DYRK (dual-specificity tyrosine phosphorylation-regulated) kinase Pom1, the Bud6/Aip6-related actin-/formin-interacting protein Bud6 and others to regulate growth [2] , [3] , [4] . Here we demonstrate that in fission yeast, polarity factors localize to the cellular cortex in distinct clusters, resolvable to ~50–100 nm in size with a ~42.5-nm lateral resolution limit. We show that oligomerization can lead to clustering and cortical enrichment of polarity factors in cells, indicating it as a possible causative mechanism for cluster formation and function. We also show that different polarity factors are segregated in different clusters at the cell cortex. Importantly, we show that for the polarity factors Tea1 and Tea3 this segregation may be key to allow cells to control polarity through the cell cycle, in particular the proper reactivation of polarized growth after mitosis. Thus, spatial segregation of polarity factor clusters provides a means to spatio-temporally control polarity at the cell cortex in this species. As we observe similar polarity factor clusters in Saccharomyces cerevisiae and Caenorhabditis elegans cells, the clustered organization of polarity factors within cortical subdomains and regulated cluster segregation may be key regulatory features across many organisms. Polarity factors localize to discrete cortical clusters To clarify the higher-order organization of the S. pombe polarity machinery, we sought to image its cortical distribution with the best possible resolution. To this end, we combined a new imaging protocol, whereby live cells are filmed frontally or ‘head-on’ rather than laterally (the way fission yeast cells are typically filmed), with high-resolution wide-field and super-resolution microscopy. In laterally imaged cells, a functional fusion of Tea1 to green fluorescent protein (GFP) expressed at the endogenous level contiguously decorated the cell end apex, as previously shown [6] , [7] . By contrast, ‘head-on’ imaging of cell ends revealed that Tea1-GFP accumulates in distinct clusters (‘nodes’) at the cell end cortex ( Fig. 1a ). Tea1 possesses a putative trimerization domain, and a theoretical model based on FRAP (Fluorescence Recovery After Photobleaching) data has suggested that Tea1 forms oligomers at the cortex [8] , a feature that could be compatible with it also forming nodes. However, we found that nodular organization was not exclusive to Tea1. Rather and strikingly, all fluorescent protein-tagged polarity factors that we imaged, including Pom1-GFP (recently reported to form aggregating and fragmenting clusters along the cell sides [9] ), Tea3-GFP, Tea4-GFP, GFP-Mod5 and Bud6-3GFP, were clearly, similarly organized in discrete cortical nodes at cell ends ( Fig. 1b ). A quantitation of node number in Tea1-GFP, Tea3-GFP, Tea4-GFP and GFP-Mod5 cells showed that a typical cell end consistently organizes 20–30 nodes of each protein dispersed along the cell cortex ( Fig. 1c ; n =10 cells), of apparently regular protein composition (of comparable fluorescence intensity). Nodularity was not due to an artifact of the fluorescent protein tag fused to polarity factors, as endogenous untagged Tea1 also localized to nodes in cells by immunofluorescence and nodes were also visible in cells where polarity factors were tagged with monomeric GFP ( Fig. 1d and Supplementary Fig. S1a ). Intriguingly, nodes did not appear to correspond to similarly distributed lipid microdomains, as neither the localization of the ergosterol-binding chemical Filipin [10] nor that of a GFP-fusion with the membrane-targeting CaaX motif of K-Ras (GFP-CaaX) resembled that of nodes ( Fig. 1e ). 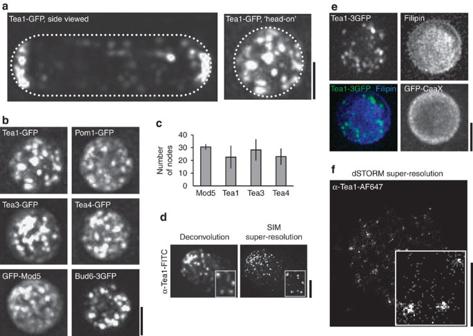Figure 1: Polarity factors localize to discrete cortical clusters (‘nodes’). (a) ‘Head-on’ versus lateral imaging of Tea1-GFP at the cell ends. (b) Examples of polarity factors forming nodes at the cell ends. (c) Average number of nodes per typical cell end for different polarity factors (n>20 cell ends). (d) Structured illumination imaging of α-Tea1-FITC nodes in an oblique oriented cell. Insets show a fourfold magnified area of the images. (e) GFP-CaaX and ergosterol (stained with Filipin) are homogeneously distributed at the cell ends. (f) Single focal plane, dSTORM microscopy imaging of α-Tea1-AF647 nodes. Inset shows a fourfold magnified area of the image. Images ina,b,dandeare maximum intensity projections of three-dimensional-deconvolved, wide-field z-stacks taken on an OMX microscope with the exception of the Filipin images, which were taken on a DeltaVision microscope. Scale bar, 2 μm. Error bars represent standard deviations. Figure 1: Polarity factors localize to discrete cortical clusters (‘nodes’). ( a ) ‘Head-on’ versus lateral imaging of Tea1-GFP at the cell ends. ( b ) Examples of polarity factors forming nodes at the cell ends. ( c ) Average number of nodes per typical cell end for different polarity factors ( n >20 cell ends). ( d ) Structured illumination imaging of α-Tea1-FITC nodes in an oblique oriented cell. Insets show a fourfold magnified area of the images. ( e ) GFP-CaaX and ergosterol (stained with Filipin) are homogeneously distributed at the cell ends. ( f ) Single focal plane, dSTORM microscopy imaging of α-Tea1-AF647 nodes. Inset shows a fourfold magnified area of the image. Images in a , b , d and e are maximum intensity projections of three-dimensional-deconvolved, wide-field z-stacks taken on an OMX microscope with the exception of the Filipin images, which were taken on a DeltaVision microscope. Scale bar, 2 μm. Error bars represent standard deviations. Full size image Three-dimensional structured illumination super-resolution microscopy (SIM) revealed that the larger looking nodes comprised multiple smaller ones and resolved nodes to a typical diameter of ~120 nm (the limit of resolution of our instrument), with each node likely containing tens of each protein (see Methods). Single focal plane direct stochastic optical reconstruction microscopy (dSTORM) with a lateral resolution limit of around 42.5 nm allowed us to resolve nodes to ~75.3±19.5 nm in diameter ( n =83 clusters), providing an upper bound of ~100 nm for node size ( Fig. 1f and Supplementary Fig. S1b ). Clusters can form and concentrate cortically by oligomerization Time-lapse fluorescence microscopy of cells expressing GFP-labelled Tea1, Tea3, Tea4 or Mod5 revealed that their nodes remained as individual entities at the cell cortex for several minutes ( Fig. 2a and Supplementary Movies 1 and 2 ), confirming that polarity nodes are persistent, dynamic structures. How could such discrete protein clusters arise and persist at the cortex? In the case of Tea1, individual nodes were seen delivered by mCherry-α-tubulin 2 (mCh-Atb2)-labelled microtubules [6] , [8] to the cortex ( Fig. 2b , top, and Supplementary Movie 3 ). There, they were subsequently retained in a Mod5-dependent manner [11] and co-localized with Mod5 nodes dynamically ( Fig. 2b , bottom, and Supplementary Movies 4 and 5 ). 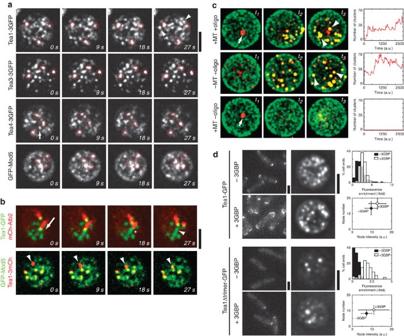Figure 2: Cortical polarity factor nodes are persistent and dynamic structures that become cortically enriched by oligomerization. (a) Time-lapse image sequences of Tea1-3GFP, Tea3-3GFP, Tea4-3GFP and GFP-Mod5. Dotted circles indicate nodes that persist through the image sequences as distinct structures; arrowheads/small arrow indicate nodes that appear/disappear, respectively. (b) Time-lapse image sequences of cells co-expressing Tea1-GFP with mCh-Atb2, and Tea1-3mCh with GFP-Mod5. In the Tea1-GFP with mCh-Atb2 sequence, a growing mCh-labelled microtubule plus end is seen delivering and leaving behind an individual Tea1-GFP node (downward arrow) that persists at the cell end cortex following microtubule catastrophe (star) and shrinkage. In the Tea1-3mCh with GFP-Mod5 sequence, an arrow indicates delivery of a Tea1-3mCh node and subsequent co-localization with a GFP-Mod5 node. (c) A computer simulation of oligomeric and microtubule-delivered (top), oligomeric and uniformly delivered (middle) and monomeric (bottom) Tea1-like polarity factors (red) interacting with a Mod5-like monomeric polarity anchor (green) constrained on a two-dimensional hemispherical cell end. Yellow indicates co-localization of Tea1 and Mod5 clusters formed. (d) Top, co-expression of a 3GBP-mCh protein enhances oligomerization of Tea1-GFP in cells, causing an increase in Tea1-GFP cell end fluorescence enrichment (n=170 side-viewed cells quantitated, top right) and node number and intensity (n=26 ‘head-on’ cells quantitated, bottom right); Bottom, oligomerization by 3GFP-mCh of a Tea1Δtrimer-GFP mutant, lacking the endogenous trimerization domain of Tea1, enhances its capacity to cluster (n=21 ‘head-on’ cells quantitated, bottom right) and restores its capacity to be cortically retained and cell end enriched (n=90 side-viewed cells quantitated, top right). Head-on cell images ina,banddare maximum intensity projections of three-dimensional-deconvolved, wide-field z-stacks taken on the OMX microscope. Side-viewed cell images indare sum projections taken on the DeltaVision microscope. Scale bar, 2 μm. Error bars represent standard deviations. Figure 2: Cortical polarity factor nodes are persistent and dynamic structures that become cortically enriched by oligomerization. ( a ) Time-lapse image sequences of Tea1-3GFP, Tea3-3GFP, Tea4-3GFP and GFP-Mod5. Dotted circles indicate nodes that persist through the image sequences as distinct structures; arrowheads/small arrow indicate nodes that appear/disappear, respectively. ( b ) Time-lapse image sequences of cells co-expressing Tea1-GFP with mCh-Atb2, and Tea1-3mCh with GFP-Mod5. In the Tea1-GFP with mCh-Atb2 sequence, a growing mCh-labelled microtubule plus end is seen delivering and leaving behind an individual Tea1-GFP node (downward arrow) that persists at the cell end cortex following microtubule catastrophe (star) and shrinkage. In the Tea1-3mCh with GFP-Mod5 sequence, an arrow indicates delivery of a Tea1-3mCh node and subsequent co-localization with a GFP-Mod5 node. ( c ) A computer simulation of oligomeric and microtubule-delivered (top), oligomeric and uniformly delivered (middle) and monomeric (bottom) Tea1-like polarity factors (red) interacting with a Mod5-like monomeric polarity anchor (green) constrained on a two-dimensional hemispherical cell end. Yellow indicates co-localization of Tea1 and Mod5 clusters formed. ( d ) Top, co-expression of a 3GBP-mCh protein enhances oligomerization of Tea1-GFP in cells, causing an increase in Tea1-GFP cell end fluorescence enrichment ( n =170 side-viewed cells quantitated, top right) and node number and intensity ( n =26 ‘head-on’ cells quantitated, bottom right); Bottom, oligomerization by 3GFP-mCh of a Tea1Δtrimer-GFP mutant, lacking the endogenous trimerization domain of Tea1, enhances its capacity to cluster ( n =21 ‘head-on’ cells quantitated, bottom right) and restores its capacity to be cortically retained and cell end enriched ( n =90 side-viewed cells quantitated, top right). Head-on cell images in a , b and d are maximum intensity projections of three-dimensional-deconvolved, wide-field z-stacks taken on the OMX microscope. Side-viewed cell images in d are sum projections taken on the DeltaVision microscope. Scale bar, 2 μm. Error bars represent standard deviations. Full size image This suggested that localized microtubule delivery (of Tea1) and/or oligomerization could suffice for the formation and maintenance of cortical nodes of both Tea1 and its interactor Mod5. To test this, we performed computer simulations of ‘Mod5-like’ molecules diffusing on a hemispherical two-dimensional cell cortex, capable of reciprocally retaining ‘Tea1-like’ molecules. When ‘Tea1’ molecules were delivered at localized points of the cortex in a microtubule-like manner and possessed an oligomerization property, this simple set of rules was sufficient to give rise in silico to assembly of a stable number of ‘Tea1’ and, indirectly, ‘Mod5’ clusters ( Fig. 2c , top, and Supplementary Movie 6 ). Similarly, localized clustering occurred even if ‘Tea1’ was homogeneously delivered to the cortex without microtubule-like events ( Fig. 2c , middle, and Supplementary Movie 6 ). By contrast, lack of oligomerization completely abolished cluster formation even if localized microtubule delivery of ‘Tea1’ packets took place ( Fig. 2c , bottom, and Supplementary Movie 6 ), demonstrating that oligomerization was indispensable for cluster formation. Hence, oligomerization could at least in part underpin the dynamical assembly and retention of Tea1 and Mod5 nodes in cells. More generally, such a mechanism could underlie the observed clustering of other polarity factors, either by virtue of their innate oligomerization capacity or indirectly via their interaction with oligomerizing factors. Importantly, although simulations could lead to the formation of discrete clusters over a large range of parameters, for many parameter values, clusters failed to form ( Supplementary Fig. S2a ). This suggests that the assembly and persistence of discrete, separate (homo- and hetero-) clusters is not an obligate consequence of oligomerization, but might instead be tightly regulated in vivo . To test the role of oligomerization in cluster formation experimentally, we generated a tandem 3GBP (GFP-Binding Protein) [12] construct capable of binding up to three GFP-labelled proteins in cells. When co-expressed with otherwise cytosolic 3GFP (not shown), 3GBP-CaaX led to the formation of 3GFP clusters throughout the cell cortex ( Supplementary Fig. S2b ), demonstrating that 3GBP can trigger GFP-labelled protein oligomerization in vivo . When co-expressed with Tea1-GFP, 3GBP led on average to the assembly of a higher number of brighter (that is, more populated; P <0.02, Student’s t -test) Tea1 clusters at and around the cell cortex area and to enhanced Tea1 cell end enrichment ( Fig. 2d , top). We then turned to a mutant form of Tea1 lacking its predicted trimerization domain (Tea1Δtrimer [8] ), which also lacks any significant cell end enrichment ( P <0.01; data not shown). In frontally viewed cells, Tea1Δtrimer-GFP assembled very few, faint (that is, very little Tea1-populated) cortical nodes following its apparently normal delivery by microtubules ( Fig. 2d , bottom, and data not shown), suggesting that in this mutant form of Tea1, the diminished oligomerization capacity is insufficient to sustain cell end enrichment. Strikingly, when co-expressed with Tea1Δtrimer-GFP, 3GBP not only induced the formation of brighter ( P <0.05) Tea1Δtrimer nodes but also restored its capacity to be cortically retained and cell end enriched ( Fig. 2d , bottom). Thus, oligomerization can trigger cluster formation and enable cortical enrichment of polarity factors in cells. Different polarity clusters co-exist on the cell cortex We next asked whether the various polarity factors localize to the same node populations, by systematically co-expressing pairs of fluorescently labelled factors in cells ( Fig. 3a ). To quantitate the spatial correlation between the different types of fluorescent nodes, we employed a point process-based spatial statistics framework that we recently developed for this purpose [13] . The framework uses Monte Carlo hypothesis testing to probe for complete spatial independence between two node populations, and a bootstrap-based statistical test to look for a significant difference in the co-localization of different pairs of node populations ( Supplementary Fig. S3 ). In the cases of Tea1 and Tea4, Tea1 and Mod5, and Tea3 and Mod5, we found that their node populations visibly co-localized and spatially correlated at short distances with high statistical significance ( Fig. 3a ). This was consistent with the fact that Tea1 and Tea4 co-immunoprecipitate in vitro [6] and that likewise Tea1, Tea3 and Mod5 co-immunoprecipitate in vitro and are all co-dependent on each other for their cortical retention at cell ends [5] . However and surprisingly, Tea1 and Tea3 nodes hardly appeared to visibly co-localize ( Fig. 3a , middle panels) and they spatially correlated more weakly (significantly less ( P <0.01) than Tea1–Tea4; see also Fig. 3c ), suggesting that Tea1 and Tea3 localize to nearby but likely distinct polarity complexes that may interact only transiently, partially or indirectly (see also Fig. 3d and Supplementary Movie 7 ). Similarly, though Pom1 localization at cell ends is Tea1- (and Tea4-) dependent [14] , [15] , Pom1 and Tea1 (and hence likely Pom1 and Tea4) also co-localized infrequently and their signals spatially correlated weakly (again significantly less ( P <0.01) than Tea1–Tea4), and Arp3 patches and Tea1 nodes did not appear to spatially correlate at all (Arp3 is an actin nucleator part of the Arp2/3 complex [16] , [17] ). Hence, multiple polarity complexes co-exist in parallel at the cell cortex during growth. 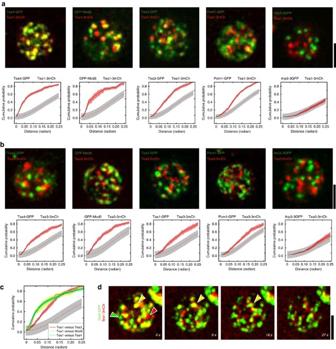Figure 3: Distinct polarity clusters co-exist on the cell cortex. Tea1-3mCh (a) and Tea3-3mCh (b) co-localization with GFP-labelled polarity factors at cell ends. Graphs represent the cumulative distribution of the distance of mCh nodes to the nearest neighbouring GFP node. Black lines within the graphs show the measured values in experimental data, with the red-shaded area showing the estimated 95% bootstrap confidence band. Red-spotted lines correspond to measurement from truly random simulated data showing no correlation across channels. The grey region indicates the range of data that would be considered random with aP=0.05 significance. (c) Comparison of Tea1-3mCh spatial correlation with Tea3-GFP, Tea4-GFP and GFP-Mod5. Tea1 is significantly more spatially correlated with Tea4 and Mod5 than Tea3 (P<0.01). (d) Time-lapse image sequence of a cell co-expressing Tea1-3mCh with Tea3-GFP. Green and red arrows indicate Tea3-GFP and Tea1-3mCh nodes non co-localizing, respectively, and the yellow arrows indicate persistent node co-localization over time. Images ina,banddare maximum intensity projections of three-dimensional-deconvolved, wide-field z-stacks taken on the OMX microscope. Scale bar, 2 μm. Figure 3: Distinct polarity clusters co-exist on the cell cortex. Tea1-3mCh ( a ) and Tea3-3mCh ( b ) co-localization with GFP-labelled polarity factors at cell ends. Graphs represent the cumulative distribution of the distance of mCh nodes to the nearest neighbouring GFP node. Black lines within the graphs show the measured values in experimental data, with the red-shaded area showing the estimated 95% bootstrap confidence band. Red-spotted lines correspond to measurement from truly random simulated data showing no correlation across channels. The grey region indicates the range of data that would be considered random with a P =0.05 significance. ( c ) Comparison of Tea1-3mCh spatial correlation with Tea3-GFP, Tea4-GFP and GFP-Mod5. Tea1 is significantly more spatially correlated with Tea4 and Mod5 than Tea3 ( P <0.01). ( d ) Time-lapse image sequence of a cell co-expressing Tea1-3mCh with Tea3-GFP. Green and red arrows indicate Tea3-GFP and Tea1-3mCh nodes non co-localizing, respectively, and the yellow arrows indicate persistent node co-localization over time. Images in a , b and d are maximum intensity projections of three-dimensional-deconvolved, wide-field z-stacks taken on the OMX microscope. Scale bar, 2 μm. Full size image Polarity cluster segregation is key for polarity control What could be the physiological advantages of spatially confining polarity regulators to nodes? One possibility is that nodes could provide a means for cells to control polarity at the cortex in space or in time, by regulating or preventing polarity factor interaction, or by segregating certain node populations from others. We tested this possibility by forcing the interaction between Tea1 and Tea3 using the GFP GBP pair [12] . We therefore engineered yeast strains co-expressing a Tea1-GBP-mCh fusion and either cytoplasmic GFP alone or Tea3-GFP. In control experiments, where cells co-expressed Tea1-GBP-mCh and GFP, Tea1 recruited GFP to nodes at the cell end cortex, and cells grew and divided indistinguishably from wild-type cells ( Fig. 4a , left, and data not shown). As expected, in cells co-expressing Tea1-GBP-mCh and Tea3-GFP, Tea3 and Tea1 nodes visibly strongly co-localized ( Fig. 4a , right). Strikingly, in those cells, the Tea1-Tea3 node populations remained at the cell cortex over relatively long time periods and became gradually displaced from the cell end cortex to the cell side cortex ( Supplementary Movie 8 ), implying that spatial segregation of these two factors is important for their correct cortical localization. Importantly, this resulted in a significant proportion of misshapen cells ( Fig. 4c and Supplementary Fig. S4 ). These defects were not due to the tags themselves, as cells expressing Tea1-GBP-mCh or Tea3-GFP separately did not display such severe defects nor were their nodes displaced from the cell ends in those cells (data not shown). Also, co-expression of Tea1-GBP and Tea4-GFP, which naturally co-localize, did not result in a morphological defect ( Figs 4b and c ), confirming that this defect was due to induced co-localization of Tea1 specifically with Tea3. Similarly, lateral mislocalization of Tea1 and Tea3 nodes and a high proportion of misshapen cells were observed in cells expressing a genetic fusion of Tea1 and Tea3 ( Supplementary Fig. S5 ). Thus, despite their nearby cortical accumulation, Tea1 and Tea3 require to be able to belong to spatially distinct node populations to properly regulate polarized growth. 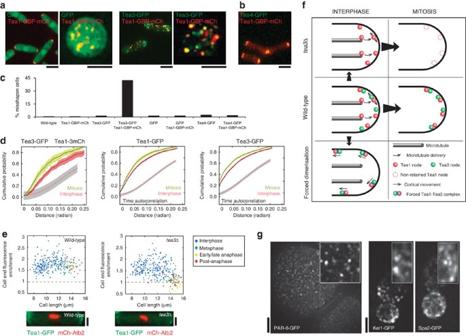Figure 4: Spatial clustering of polarity complexes is key for their proper function and may be a ubiquitous regulatory feature. (a) Dimerization of Tea1-GBP-mCh and Tea3-GFP in cells causes close co-localization of Tea1 and Tea3 nodes and affects their cortical localization. This does not happen upon dimerization of Tea1-GBP-mCh with cytoplasmic GFP, where Tea1 and GFP co-localize normally in nodes, at the cell ends. Cells expressing cytoplasmic GFP alone in absence of Tea1-GBP-mCh do not assemble GFP clusters at cell ends (data not shown). (b) Forced dimerization of Tea4-GFP with Tea1-GBP-mCh does not disrupt their localization. (c) Percentage of the cell population displaying a misshapen phenotype for Tea1-GBP-mCh and Tea3-GFP expressing cells, compared with different control cells (n≥100 cells for each case). (d) Co-localization of Tea1-3mCh and Tea3-GFP nodes at cell ends is stronger in mitosis than in interphase (n=20 cells for each case); cell-cycle stage was monitored by co-expressing in cells the B-cyclin Cdc13-GFP. The dynamics of Tea1-GFP (Tea1-GFP, left) and Tea3-GFP (Tea3-GFP, right) nodes is lower in mitosis than in interphase cells (P<0.01), as assessed by quantitating the nodes’ auto-correlation between timetand timet+3 s for multiple, consecutive time-lapse images. Cell-cycle stage was monitored by co-expressing in cells mCh-Atb2. (e) Tea1-GFP fluorescence enrichment at the cell ends is consistent throughout the cell cycle in wild-type cells, but is lost specifically in mitotic cells lacking Tea3. Cell-cycle stage was monitored by co-expressing in cells the microtubule marker mCh-Atb2 (n>650 cells). (f) Schematic model of Tea1/Tea3 interactions through the cell cycle. (g) PAR-6-GFP clusters observed in a live two-cell stageC. elegansembryo (left), and Kel1-GFP and Spa2-GFP clusters observed inS. cerevisiaecells (right). Images of head-on cells inaand images ingare maximum intensity projections of three-dimensional-deconvolved, wide-field z-stacks taken on the OMX microscope, and images of side-on cells ina,bandeare maximum intensity projections of wide-field z-stacks taken on the DeltaVision. Scale bar, 2 μm with exception of theC. elegansimage where it represents 20 μm. Figure 4: Spatial clustering of polarity complexes is key for their proper function and may be a ubiquitous regulatory feature. ( a ) Dimerization of Tea1-GBP-mCh and Tea3-GFP in cells causes close co-localization of Tea1 and Tea3 nodes and affects their cortical localization. This does not happen upon dimerization of Tea1-GBP-mCh with cytoplasmic GFP, where Tea1 and GFP co-localize normally in nodes, at the cell ends. Cells expressing cytoplasmic GFP alone in absence of Tea1-GBP-mCh do not assemble GFP clusters at cell ends (data not shown). ( b ) Forced dimerization of Tea4-GFP with Tea1-GBP-mCh does not disrupt their localization. ( c ) Percentage of the cell population displaying a misshapen phenotype for Tea1-GBP-mCh and Tea3-GFP expressing cells, compared with different control cells ( n ≥100 cells for each case). ( d ) Co-localization of Tea1-3mCh and Tea3-GFP nodes at cell ends is stronger in mitosis than in interphase ( n =20 cells for each case); cell-cycle stage was monitored by co-expressing in cells the B-cyclin Cdc13-GFP. The dynamics of Tea1-GFP (Tea1-GFP, left) and Tea3-GFP (Tea3-GFP, right) nodes is lower in mitosis than in interphase cells ( P <0.01), as assessed by quantitating the nodes’ auto-correlation between time t and time t +3 s for multiple, consecutive time-lapse images. Cell-cycle stage was monitored by co-expressing in cells mCh-Atb2. ( e ) Tea1-GFP fluorescence enrichment at the cell ends is consistent throughout the cell cycle in wild-type cells, but is lost specifically in mitotic cells lacking Tea3. Cell-cycle stage was monitored by co-expressing in cells the microtubule marker mCh-Atb2 ( n >650 cells). ( f ) Schematic model of Tea1/Tea3 interactions through the cell cycle. ( g ) PAR-6-GFP clusters observed in a live two-cell stage C. elegans embryo (left), and Kel1-GFP and Spa2-GFP clusters observed in S. cerevisiae cells (right). Images of head-on cells in a and images in g are maximum intensity projections of three-dimensional-deconvolved, wide-field z-stacks taken on the OMX microscope, and images of side-on cells in a , b and e are maximum intensity projections of wide-field z-stacks taken on the DeltaVision. Scale bar, 2 μm with exception of the C. elegans image where it represents 20 μm. Full size image We therefore wondered whether the spatial segregation of Tea1 and Tea3 nodes could be important for cells to undergo any of the major transitions in their polarized growth pattern, during the cell cycle. Using cells co-expressing Tea1-YFP, Tea3-3mCh and the Arp2/3 component Arp2-CFP (which localizes to actin patches and is enriched in growing cell ends [18] ), we found no statistical difference in the spatial correlation between Tea1 and Tea3 in growing versus non-growing cell ends, implying that the segregation of Tea1 from Tea3 nodes likely does not have a role in the transition from monopolar to bipolar growth ( Supplementary Fig. S6 ). By contrast, when we looked at cells co-expressing Tea1-3mCh, Tea3-GFP and a reporter of cell-cycle stage, such as the B-type cyclin Cdc13-GFP [19] ( Fig. 4d , left, and Supplementary Fig. S7a ) or the spindle pole body component Alp6-GFP [20] ( Supplementary Figs S7b and S7c and Supplementary Movies 9 and 10 ), we found a significant ( P <0.01) increase in the spatial correlation of Tea1 and Tea3 nodes specifically in mitosis compared with interphase. This coincided with a significantly increased ( P <0.01) temporal auto-correlation of Tea1/Tea3 nodes with themselves specifically in mitosis ( Fig. 4d , middle and right), suggesting that the cortical dynamics of both protein nodes decreases, probably as a consequence of their increased co-localization, and that both protein nodes likely physically interact during mitosis. To test this further, we quantitated the enrichment at cell ends of Tea1 or Tea3 in cells knocked out for tea3 ( tea3Δ ) or tea1 ( tea1Δ ), respectively, and found that, although Tea3 cell end enrichment was unaffected in tea1Δ cells (not shown), Tea1 enrichment was completely abolished at tea3Δ cell ends specifically in mitosis ( Fig. 4e ). Furthermore, Tea1 enrichment at the cell ends was also abolished in tea3Δ cells arrested in a prolonged mitosis, but not in wild-type cells ( Supplementary Fig. S8 right and left, respectively). We conclude that increased co-localization of Tea1 and Tea3 nodes may be needed to secure the continued cell end retention of the Tea1 growth landmark during mitosis, when the cytoplasmic microtubule system is disassembled and can no longer sustain Tea1 cell end enrichment. As both tea3Δ and tea1Δ cells have severe defects in resuming growth from their old ends following mitosis [21] , this in turn may be key for the proper reactivation of polarized growth following cell division. A schematic model summarizing these results is shown in Fig. 4f . In wild-type interphase cells, Tea1 is delivered by microtubules, and Tea1 nodes spatially correlate only weakly with Tea3 nodes at the cell cortex. During mitosis, microtubule delivery of Tea1 nodes ceases and there is a closer spatial correlation between Tea1 and Tea3. In tea3Δ cells, Tea1 nodes are retained during interphase but not in mitosis, suggesting that Tea3 retains Tea1 in the absence of microtubule delivery. Forced dimerization of Tea1 and Tea3 prevents segregation of their nodes and causes the prolonged retainment at the cortex of Tea1 nodes, which become laterally displaced along the cortex because of a lack of Tea1 cortical turnover and re-delivery by microtubules. Altogether, our results suggest that regulated cortical clustering is key to spatio-temporal control of cell polarity in fission yeast. To determine if this paradigm could extend beyond fission yeast, we imaged with similar resolution related polarity factors in the budding yeast S. cerevisiae and the nematode C. elegans . Remarkably, similar persistent cortical clusters of the polarity regulators PAR-6-GFP [22] ( Fig. 4g , left, and Supplementary Movie 11 ) and Kel1-GFP and Spa2-GFP [23] , [24] ( Fig. 4g , right, and Supplementary Movies 12 and 13 ) could be observed in C. elegans and S. cerevisiae cells, respectively. Hence, we extrapolate that regulated clustering and segregation of polarity proteins could represent a common organizational principle in a wide range of cell types and organisms. In summary, the polarity machinery of fission yeast is arranged into cortical clusters that are dynamic and persistent, and may be formed by oligomerization (direct or mediated by an interacting partner). Many polarity factors can be found in neighbouring but separate cluster populations, with this spatial segregation potentially key to their function. Although the clusters are dynamic, they are also persistent and appear relatively immobile ( Fig. 2a ), and it is not yet clear what the functional significance of that persistence/immobility might be. One possibility is that it may allow polarity factors to maintain a stable domain of localization and function. Alternatively, it may ensure that certain polarity factor clusters only interact with others at specific locations and times within the cell, as exemplified by Tea1 and Tea3 ( Fig. 4d , left). This suggests that the interaction between different polarity factor species may be an actively regulated feature, and not simply occur as a default when polarity factors reside within a same general domain at the cell cortex. Future work should aim to clarify how the various polarity factors are targeted to different clusters. This may be accomplished through post-translational modification of certain polarity factors [25] , [26] , through competitive binding interactions (for example, with a common cortical anchor such as Mod5 (ref. 5 )) that could cause cluster segregation, or via other mechanisms. Although the widespread clustered organization of the polarity machinery described here had never been demonstrated before, cortical protein clusters have been observed in other contexts. For instance, in fission yeast cells, multi-protein medial cortical nodes—whose yet unexplained clustered formation is initiated by phosphorylation of the oligomeric anillin Mid1 [27] , [28] and which recruit sequentially factors like the Wee1-inhibiting protein kinase Cdr2 and Myosin II—are thought to regulate cell size-dependent mitotic onset and, subsequently, activation of contractile acto-myosin ring formation during cytokinesis [28] , [29] , [30] . In budding yeast cells, GTP-Cdc42 localizes to stochastically arising clusters that become amplified during cell polarization [31] , and plasma-membrane-bound proteins are organized in patterns that range from cluster-like patches to semi-continuous networks depending on the transmembrane sequences they possess [32] . In C. elegans , the conserved PDZ domain-containing protein PAR-3, which acts together with PAR-6 and PKC-3 (atypical protein kinase) to regulate cell polarity, self-oligomerizes via its CR1 domain to achieve its cortical distribution and function during early embryogenesis [33] . And in mammalian cells, the SNARE-family syntaxin 1 protein, which defines sites at which secretory granules fuse, self-organizes homo-oligomers via its SNARE motif [34] , and Ras GTPase nanoclusters are thought to act as high-fidelity membrane-bound signal transducers in the Ras–Raf–MEK–ERK kinase signalling cascade, effectively functioning as nano-switches [35] , [36] , [37] . Thus, cortical compartmentalization of proteins into discrete clustered domains may be a general feature exploited by cells to control spatiotemporal signalling events with high fidelity [38] . In the case of cell polarity, cortical nodes and their spatial segregation could contribute to robust ‘on’ or ‘off’ switching of polarity at the right place and time in cells, following intra- or extracellular signals. As deregulation of polarity has been implicated in many diseases, including cancer [39] , future work should investigate whether frequent mutations exist that do not affect the individual characteristics of polarity factors but specifically perturb or induce their capacity to cluster, and the relevance of those mutations to disease. S. pombe strains and plasmid construction The S. pombe strains used in this study are listed in Supplementary Table S1 . Conventional PCR-based gene targeting methods for S. pombe were used for gene tagging [40] , [41] and are described further in the Supplementary Information . Frontal imaging of S. pombe cells Before imaging, S. pombe strains were grown at 32 °C in yeast extract with supplements (YES) [42] to exponential growth with the exception of nmt81-GFP-Mod5 strains and strain RCS460 (GFP-CaaX), which were grown at 32 °C in minimal medium (EMM) [42] overnight. Aliquots of 300 μl cells were mounted onto 1.5 coverslip glass-bottom plastic dishes (MatTek; P35G-1.5-14-C) pre-coated with 10 μl 1 mg ml −1 lectin (Sigma; L1395 and Patricell Ltd; L-1301-25) that had been allowed to air dry. After a 30-min incubation, cells unbound to the lectin-coated glass were removed by washing with EMM, and bound cells were kept in a final suspension of 1 ml EMM. Bound cells found to be frontally arrayed (‘head-on’) were then visually selected for imaging. ‘Head-on’ imaging of vertically arrayed cells unless otherwise stated was performed on an OMX microscope (Applied Precision) in conventional resolution mode, with an Olympus UPlanSapo × 100 oil immersion lens (numerical aperture 1.4) and 1.512 refractive index immersion oil (Applied Precision). That system allows for superior imaging than an equivalent wide-field microscope with a × 100 1.4 numerical aperture lens even in conventional mode, due to its very low levels of non-Poisson noise, multiple ultra-sensitive EMCCD cameras and a very stable, accurate and quick stage for the creation of z-stacks. z-stacks of ‘head-on’ cell ends were imaged at 0.125 μm intervals over 17 focal planes and deconvolved and analysed using SoftWoRx. GFP and mCherry fluorophores were imaged with 488 and 594 nm laser lines, respectively, with the standard filter sets. CFP, YFP in combination with mCherry fluorophores, were imaged with 405, 514 and 594 nm laser lines, respectively, with the live-cell filter set. Multi-colour images were taken in sequential mode and corrected for chromatic aberration using SoftWoRx. Time-lapse images were taken at the time intervals stated. For ‘head-on’ imaging of cell ends in combination with cell-cycle stage determination, first short 17 focal plane stacks at 0.125 μm intervals were taken of the cell ends followed by longer 144 plane stacks at 0.125 μm intervals of the whole cell, which were then reconstructed in the Volume Viewer function of SoftWoRx. Cell cycle stage reporters were Cdc13-GFP (B-cyclin), Alp6-GFP (a γ-tubulin complex component localized to the spindle pole body) or mCh-Atb2 (α-tubulin 2), as specified in the Figures. Estimation of the number of polarity factors per node was as follows. It has been established (Bicho et al . [8] ) by lateral imaging that a typical fission yeast cell contains ~8,000 Tea1 molecules, a typical cell end contains ~1,500 Tea1 molecules and an individual Tea1 packet delivered by microtubules to the cell end cortex consists of ~80 molecules. As shown here, Tea1 packets delivered to the cortex were subsequently retained there as nodes ( Fig. 2b and Supplementary Movie 3 ), maintaining a similar fluorescence intensity (data not shown). Hence, a typical Tea1 node viewed in conventional wide-field deconvolved images comprised likely a similar number of proteins (~80). We corroborated this number by calculating the proportion of the total cell fluorescence corresponding to cell ends (~40%=2*20% per cell end) and dividing it by the total number of nodes at cell ends (~50=2*25 per cell end). Thus, the average number of Tea1 proteins per node is: 8,000*0.40/50=~64 Tea1 proteins. Similarly, we compared the total fluorescence intensity of cells expressing Tea3-GFP and Tea4-GFP with that of cells expressing Tea1-GFP to estimate the total number of Tea3 and of Tea4 proteins in cells; subsequently, based on the average number of Tea3/Tea4 nodes at cell ends, we approximated the average number of Tea3 and Tea4 proteins per node to be also ~50 Tea3/Tea4 proteins per node. Thus, a typical polarity factor cluster contains likely tens of proteins. Structured illumination super-resolution imaging For SIM imaging, cells of the wild-type S. pombe strain 972 were stained with Anti-Tea1-FITC antibody as described previously [7] . Stained cells were pipetted onto 1.5 cm coverslip glass-bottom plastic MatTek dishes and kept immobile by setting in hand-cooled molten 1% low-melting point agar (Invitrogen; 16520-050). Images of ‘head on’ cells were taken at 0.125 μm intervals over 17 planes on the OMX microscope in SIM mode. The SIM stacks were then reconstructed into final images using SoftWoRx. Based on the estimated average number of ~64 Tea1 proteins per large wide-field node (see above), and on the observation that wide-field nodes often comprise multiple (2 or 3) smaller nodes resolvable by SIM to ~120 nm ( Fig. 1d and quantitation not shown), we estimate on average ~20–30 Tea1 proteins per SIM resolvable cluster. dSTORM super-resolution imaging For dSTORM imaging, cells of the wild-type S. pombe strain 972 were stained with Anti-Tea1 and Anti-Rb-AF647 (Life Technologies A-21245) as described previously [7] . The cells were immobilized on poly-lysine-coated glass-bottom MatTek dishes and covered with STORM Imaging Buffer with MEA (Nikon Instruments, Nikon Corporation, Japan). Imaging was performed on an N-STORM superresolution imaging system (Nikon) with an × 100 oil objective and Andor iXon camera. Analysis was carried out using QuickPALM with a signal-to-noise ratio threshold of 5. Images were rendered with a 10-nm pixel size and simulated subdiffraction Gaussian spots. Estimation of the uncertainty in the measurement of fluorophore position was done by taking into consideration the size of the antibodies used (~10 nm per antibody) and the localization precision of the measurement (calculated to be ~12 nm, based on the emitted number of photons and the background in our images). This leads on average to a combined uncertainty (standard deviation, s.d.) in our measurement of fluorophore position of ~18.5 nm. Precise estimation of labelling efficiency is generally impracticable. However, given the measured range of Tea1 cluster size values observed by STORM (~50–100 nm with a median/s.d. of ~75.3±19.5 nm, n =83 clusters; Supplementary Fig. S1b ) and the Gaussian width predicted by the estimated uncertainty in our measurements (full width at half maximum (FWHM)=42.5 nm=2.3*18.5 nm), we did a two-dimensional simulation of a cluster of ~25 proteins with only a fraction of proteins labelled by a fluorophore (not shown). We found that for clusters containing 20–100% of labelled proteins, the measured cluster size would be within ~10% of its true value (FWHM and s.d. obtained from 1,000 simulation repetitions). In addition, for a cluster of 25 proteins comprising four contiguous fluorophore-labelled proteins that cannot be separated by more than 42.5 nm (or else they could be distinguished as two peaks), we found that the absolute highest measured cluster size would be ~64 nm at maximal fluorophore separation. This is less than the median cluster size measured of ~75 nm, suggesting that clusters that we observe with STORM contain on average multiple (>20%) proteins labelled, and that, therefore, our measured protein cluster size is representative of the actual cluster size. Computer simulation of cortical cluster formation Simulation of the formation of cortical polarity factor complexes was done using a particle-based framework based on the theoretical framework Smoldyn ( http://www.smoldyn.org/index.html ). All species moved by Brownian motion, and most parameter values were taken from the literature or sensibly estimated. Visual rendering of the simulations was done by applying a Gaussian convolution around simulated proteins or complexes’ positions, to emulate a microscope point spread function. Cluster detection and co-localization statistical analysis Detection of cortical polarity factor clusters (‘nodes’) was performed on three-dimensional (xyz) image stacks of cell ends of interest, using the ‘spot detector’ module of the open-source software ICY ( http://www.bioimageanalysis.org/icy/index.php ). Statistical assessment of co-localization between two different protein node populations was done using simulation-based Monte–Carlo hypothesis testing, by simulating the spatial distribution of node populations following the null hypothesis as two inhomogeneous Poisson spatial point processes drawn independently. The significance of the test was linked to the number of simulations performed, with a confidence band determined by bootstrap-based statistical testing. See Supplementary Information for Extended Materials and Methods, including further information on cortical cluster detection and statistical assessment of cluster co-localization and computer simulation of cortical cluster formation. S. cerevisiae yeast strains and imaging All S. cerevisae strains used are described in Supplementary Table S1 . Strain MGY242 was derived from strain 15D using standard genetic techniques [43] . For imaging, strains were grown to exponential phase in yeast extract peptone dextrose (YPD), and 300 μl of cells were then mounted onto 1.5 coverslip glass-bottom plastic MatTek dishes pre-coated with 10 μl Concanavalin A (Sigma) that had been allowed to air dry. After a 30 min incubation, cells unbound to the Concanavalin A-coated glass were removed by washing with yeast nitrogen base [43] , and the bound cells were kept in a final suspension of 1 ml yeast nitrogen base. C. elegans lines and imaging JJ1579 gravid C. elegans worms ((unc-119Ied3) III; zuls77 (par6-6p::PAR-6::GFP;unc-119(+))) were dissected in M9 Buffer (22 mM KH 2 PO 4 , 43 mM Na 2 HPO 4 , 85 mM NaCl and 1 mM MgSO 4 ) in a watch glass and transferred by mouth pipette onto 3% agarose pads. The embryos were compressed slightly by 18 × 18 mm 2 glass coverslips to optimize viewing. All embryos were imaged on the OMX microscope in conventional mode. How to cite this article: Dodgson, J. et al . Spatial segregation of polarity factors into distinct cortical clusters is required for cell polarity control. Nat. Commun. 4:1834 doi: 10.1038/ncomms2813 (2013).